Capacitance of carbon-based electrical double-layer capacitors Experimental electrical double-layer capacitances of porous carbon electrodes fall below ideal values, thus limiting the practical energy densities of carbon-based electrical double-layer capacitors. Here we investigate the origin of this behaviour by measuring the electrical double-layer capacitance in one to five-layer graphene. We find that the capacitances are suppressed near neutrality, and are anomalously enhanced for thicknesses below a few layers. We attribute the first effect to quantum capacitance effects near the point of zero charge, and the second to correlations between electrons in the graphene sheet and ions in the electrolyte. The large capacitance values imply gravimetric energy storage densities in the single-layer graphene limit that are comparable to those of batteries. We anticipate that these results shed light on developing new theoretical models in understanding the electrical double-layer capacitance of carbon electrodes, and on opening up new strategies for improving the energy density of carbon-based capacitors. Electrical double-layer (EDL) capacitors, also known as supercapacitors, are promising for energy storage when high power density, high cycle efficiency and long cycle life are required. Unlike batteries, which store energy in chemical bonds, EDL capacitors store electrical energy at an electrode–electrolyte interface [1] , [2] , [3] when a voltage bias is applied. The absence of the resistances associated with the charge-transfer reactions present in batteries allows the energy to be stored and delivered at extremely high power. The maximum capacitance of EDL devices is on the order of hundreds of farads per gram, orders of magnitude larger than that of a traditional dielectric capacitor whose capacitance is typically in the microfarad per gram range. Large capacitances are achievable thanks to the extremely short charge separation distance (<1 nm) at the electrode–electrolyte interface, and the exceptionally high specific surface area (SSA, 500–3,000 m 2 g −1 ) of porous carbon electrodes. The highest energy storage densities of commercially available EDL capacitors, based on high surface area activated carbons, are nevertheless still below 12 Wh kg −1 (ref. 4 ), an order of magnitude smaller than in Li-ion batteries. Research has therefore focused on increasing the energy density of EDL capacitors without sacrificing the power density and cycle life. Optimization of the electrode material is crucial, since at a given maximum voltage the total stored energy is proportional to the capacitance. A large SSA is one of the most important parameters leading to a large gravimetric capacitance and hence energy storage density [5] . Although tremendous progress has been made in increasing the SSA of carbon materials by engineering appropriate porous structures, experimentally obtained EDL capacitance of pure carbon electrodes remains lower than expected given the large SSA values. An analysis of the capacitance–surface area relationship for various pure carbon electrodes from the literature is provided in Fig. 1 (refs 6 , 7 , 8 , 9 , 10 , 11 , 12 , 13 , 14 , 15 , 16 , 17 , 18 ). There we can see that the gravimetric capacitance (F g −1 ) increases together with the SSA of the carbon electrodes but the area-normalized capacitance ( C A , μF cm −2 ) gradually decreases and stabilizes, respectively, at about 4–5 μF cm −2 when the SSA is larger than 1,500 m 2 g −1 , both at the point of zero charge (PZC) and over the whole operating voltage range. The low C A values observed in the highest SSA carbons are the main factor limiting the total achievable gravimetric capacitance in carbon-based electrodes. Numerous studies over the past decades have attempted to understand the origin of this limitation [18] , [19] , [20] , [21] , [22] . The simplest estimate of EDL capacitance in a planar system includes only electrical energy, leading to the familiar geometric capacitance expression (in units of F g −1 ): C=C A A=ε 0 ε r A/d , where ε 0 is the dielectric constant in vacuum (~8.854 × 10 −12 F m −1 ), ε r is the relative dielectric constant of the electrolyte, A is the area of electrode exposed to the electrolyte (m 2 g −1 ) and d is the charge separation distance (m). ( C A is the area-normalized capacitance of the EDL (F m −2 )) [23] . Taking the dielectric constant of most commonly used solvents such as water ( ε r is ~80.1), acetonitrile (AN, ε r is ~37.5) and propylene carbonate ( ε r is ~64) and adopting a large estimate of the average charge separation distance of 1 nm, would imply that C A is in the range of 30–70 μF cm −2 for flat surface metal electrodes. The origin of the factors which limit C A to values as low as 4~5 μF cm −2 in carbon-based electrodes remains an unresolved puzzle. 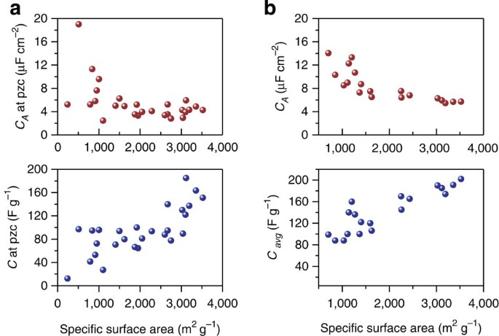Figure 1: EDL capacitance with respect to SSA of porous carbon material. (a) The area-normalized capacitance (CA, top) and the gravimetric capacitance (C, bottom) of various types of porous carbon electrodes at the PZC versus the BET SSA (SBET). (b) The average area-normalized capacitance (top) and the gravimetric capacitance (bottom) of various types of porous carbon electrodes over the entire operating potential changes with the SSA. Data are collected from the literature among those works that strictly followed the stringent supercapacitor test procedures and conditions. The electrode materials are porous carbon electrodes with no additional functionalities or dopants. The capacitances were collected at slow scan rates with near ideal CV curves to exclude the diffusion and sieving effects. Figure 1: EDL capacitance with respect to SSA of porous carbon material. ( a ) The area-normalized capacitance ( C A , top) and the gravimetric capacitance ( C , bottom) of various types of porous carbon electrodes at the PZC versus the BET SSA ( S BET ). ( b ) The average area-normalized capacitance (top) and the gravimetric capacitance (bottom) of various types of porous carbon electrodes over the entire operating potential changes with the SSA. Data are collected from the literature among those works that strictly followed the stringent supercapacitor test procedures and conditions. The electrode materials are porous carbon electrodes with no additional functionalities or dopants. The capacitances were collected at slow scan rates with near ideal CV curves to exclude the diffusion and sieving effects. Full size image In order to address this outstanding question, here we undertake a systematic study of capacitance in systems with carbon-based electrodes consisting of ultrathin graphene layer stacks. We find that the reduction in capacitance at the PZC can be attributed to graphene sheet quantum capacitance. However, our control of electrode thickness down to a single graphene layer, together with the accuracy and reproducibility of our measurements, have allowed us to experimentally identify an unexpected increase of C A with decreasing electrode thickness when the electrode is charged. As explained below, we attribute the increase to electrostatic correlations between graphene sheet electrons and electrolyte ions. More importantly, our findings point to new strategies for improving the capacitance of carbon-based electrodes. Preparation and characterization of graphene electrodes Traditional methods for preparing carbon materials do not offer precise control over relevant physical properties including morphology, curvatures, conductivities and so on, making studies of C A versus SSA rather difficult. Moreover, carbon materials prepared through different processes vary in surface chemistry that might lead to a pseudocapacitive contribution due to functional groups [24] , [25] . We overcame these difficulties by preparing planar carbon electrodes with different SSA by randomly stacking multilayer graphene and nitrogen-doped single-layer graphene sheets. We studied the EDL capacitance of these planar graphene electrodes in a 6 M potassium hydroxide aqueous electrolyte. The single-layer graphene was synthesized using chemical vapour deposition with methane and hydrogen gases on copper foil (see Methods and Supplementary Fig. 1 and Supplementary Note 1 ) [26] . As described in Fig. 2 , we prepared electrodes with different numbers of graphene layers by repeated transfer of poly(methyl methacrylate) (PMMA)-coated graphene onto a single-layer graphene-coated copper foil, and then partially dissolved the copper to expose an n -layer graphene surface without polymer residuals to the electrolyte solution. The graphene electrodes were fabricated to be rectangular with a surface area of several square millimetres ( Fig. 2 ). The SSA of flat electrodes is inversely proportional to the number of stacked layers. Scanning electron microscopy ( Supplementary Fig. 2 and Supplementary Note 2 ), Raman mapping ( Supplementary Fig. 3 and Supplementary Note 2 ) and sheet conductance tests ( Supplementary Fig. 4 and Supplementary Note 2 ) showed that the randomly stacked n -layer graphene electrode’s integrity was preserved after the transfer. This ensured good homogeneity in thickness over the entire n -layer graphene electrode. Neither faradic reaction nor ion specific adsorption occurred at the electrode surface during the cyclic voltammetry (CV) measurement ( Supplementary Fig. 5 ), indicating that the surface of the graphene electrode was clean. The CV curves remained almost unchanged after the capacitance measurements, suggesting excellent structural stability. Therefore, we can expect that (i) graphene electrodes with the planar morphology used in our study effectively exclude uncontrolled effects due to pore size, uncontrolled morphology and curvature, (ii) the surface areas of the various electrodes in contact with the electrolyte are directly measured without the Brunauer–Emett–Teller (BET) limitation and (iii) the electrodes are sp 2 -hybridized carbon without a pseudocapacitive contribution. All of the above features make our graphene electrodes ideally suited for our electrode capacitance study. 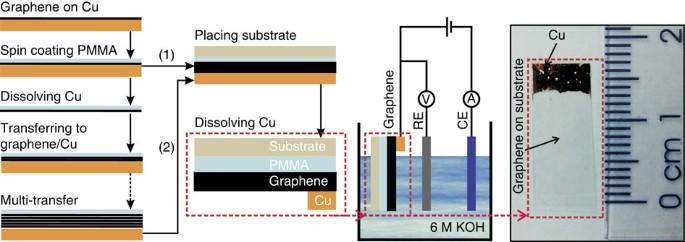Figure 2: Graphene electrode fabrication and capacitance measurement. The single-layer graphene electrode was prepared by placing a plastic substrate on a graphene coated Cu foil, and then exposing the graphene surface by partially dissolving Cu. The multilayer graphene electrodes were prepared by repeated transfers of PMMA-coated graphene films onto a single-layer graphene-coated Cu foil, placing the plastic substrate and then partially dissolving Cu. This process yielded a polymer residual-free graphene surface. The capacitance was measured with a three-electrode electrochemical cell in a 6 M KOH aqueous electrolyte. The photograph shows a graphene electrode with partially dissolved copper as the electrical contact. The surface area of the graphene electrode that is exposed in the electrolyte solution can be directly measured, avoiding possible errors due to the assumption that the BET surface area equals that of the electrode exposed to the electrolyte solution. Figure 2: Graphene electrode fabrication and capacitance measurement. The single-layer graphene electrode was prepared by placing a plastic substrate on a graphene coated Cu foil, and then exposing the graphene surface by partially dissolving Cu. The multilayer graphene electrodes were prepared by repeated transfers of PMMA-coated graphene films onto a single-layer graphene-coated Cu foil, placing the plastic substrate and then partially dissolving Cu. This process yielded a polymer residual-free graphene surface. The capacitance was measured with a three-electrode electrochemical cell in a 6 M KOH aqueous electrolyte. The photograph shows a graphene electrode with partially dissolved copper as the electrical contact. The surface area of the graphene electrode that is exposed in the electrolyte solution can be directly measured, avoiding possible errors due to the assumption that the BET surface area equals that of the electrode exposed to the electrolyte solution. Full size image EDL capacitance of graphene with layer number of 1–5 We measured the area-normalized EDL capacitance (also called the interfacial capacitance), C EDL , of the graphene electrodes at different electrode potentials using frequency response analysis (see Methods, Supplementary Fig. 6 and Supplementary Note 3 for details of the measurements). C EDL versus V EDL curves measured with 1–5-layer graphene electrodes are presented in Fig. 3a . The C EDL − V EDL curves are all concave shaped with the capacitance minimum located in the V EDL range of −0.1 to 0.15 V, indicating slight carrier doping by residue from the graphene transfer process. For each type of graphene electrode, we measured 3–7 sample devices. The mean minimum values of C EDL vary over the limited range from 2.5 to 3.5 μF cm −2 with layer number n , and are close to the values measured on the basal plane of highly oriented pyrolytic graphite (HOPG) ( Fig. 3b ) by Randin and Yeager in 1971 and Gerischer et al . in 1987, respectively [27] , [28] . On the other hand, the magnitudes of the slopes of the left and right arms of the C EDL − V EDL , which correspond to electron- and hole-doped regions, drop by about 74% when stacked graphene layer number increases from one to five, approaching values measured with HOPG ( Fig. 3c ) [27] , [28] electrodes at the thick limit. In this potential range, single-layer graphene electrodes have the largest SSA and the largest C A . 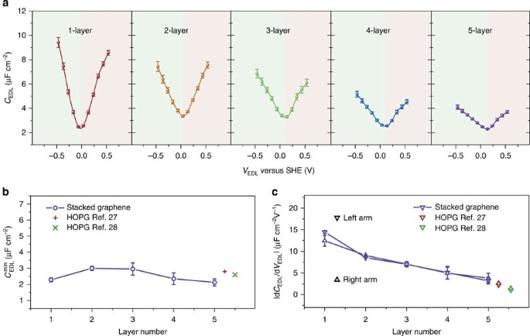Figure 3: EDL capacitance of graphene with layer numbers of 1–5. (a) EDL capacitance of graphene electrodes with different numbers of stacked single-layer graphene show a concave shape when plotted with respect to the electrode potential measured against a standard hydrogen electrode. The capacitance minimums are located in the potential range of −0.1 to 0.15 V, indicating very slight doping from graphene transfer residue contamination. The error bars are collected from the frequency response analysis and they range between 0.04 and 0.1 μF cm−2, representing the uncertainties from data processing. (b) The capacitance minimum plotted against graphene layer number. The values vary in the range of 2.5–3.5 μF cm−2independent of the number of layers and close to that measured from the basal plane of HOPG. (c) The modulus of the derivative of capacitance with respect to the graphene potential. The modulus decreases and approaches the values of HOPG with an increasing number of graphene layers. The error bars quoted inbandcoriginate reflect device-to-device variations, with uncertainties ranging between 0.13 to 0.4 μF cm−2. Figure 3: EDL capacitance of graphene with layer numbers of 1–5. ( a ) EDL capacitance of graphene electrodes with different numbers of stacked single-layer graphene show a concave shape when plotted with respect to the electrode potential measured against a standard hydrogen electrode. The capacitance minimums are located in the potential range of −0.1 to 0.15 V, indicating very slight doping from graphene transfer residue contamination. The error bars are collected from the frequency response analysis and they range between 0.04 and 0.1 μF cm −2 , representing the uncertainties from data processing. ( b ) The capacitance minimum plotted against graphene layer number. The values vary in the range of 2.5–3.5 μF cm −2 independent of the number of layers and close to that measured from the basal plane of HOPG. ( c ) The modulus of the derivative of capacitance with respect to the graphene potential. The modulus decreases and approaches the values of HOPG with an increasing number of graphene layers. The error bars quoted in b and c originate reflect device-to-device variations, with uncertainties ranging between 0.13 to 0.4 μF cm −2 . Full size image Previously small C A values on carbon electrodes have been explained by invoking a space charge capacitance [18] , [22] , [27] , [28] , representing spread of induced electrode charge into the bulk, in series with a Helmholtz capacitance C H , representing the Helmholtz layer [29] located on the liquid side of the interface, between the electrolyte and the bulk solid ( Fig. 4a ). The pronounced C A minima we observe at the PZC make it clear that this picture is incomplete. In low-dimensional materials like graphene, it is necessary to add in addition a quantum capacitance [30] , [31] C Q which accounts for the variation of Fermi energy with charge accumulated in the electrode. The quantum capacitance of graphene is small near charge neutrality due to the low density of states (DOS) near the Dirac point [30] , limiting C EDL . In multilayer electrodes, space charge and quantum capacitance effects act together to yield a modified quantum capacitance C Q defined by coupled Poisson–Schrodinger equations ( Supplementary Fig. 7 and Supplementary Note 4 ). 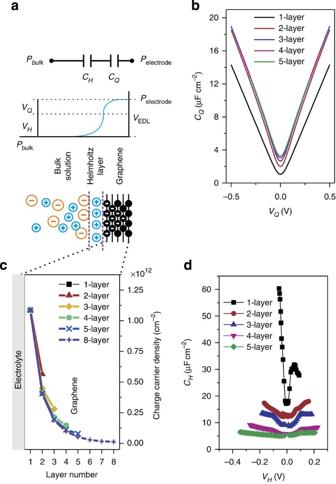Figure 4: EDL at the graphene/electrolyte interface. (a) Schematic illustration of the equivalent circuit and charge distribution near the graphene/electrolyte interface. (b) Quantum capacitance of graphene as a function of layer number and potential calculated in the standard self-consistent Hartree approximation which neglects correlations. Neglecting disorder, the carrier density in single-layer graphene is proportional to the square of the Fermi radius, and hence to square of the chemical potential. The capacitance is therefore linear in chemical potential. (c) Charge distribution induced at a potential of 0.1 V in graphene electrodes with different numbers of layers. Layer number 1 is exposed to the electrolyte. (d) Inferred Helmholtz capacitance plotted against inferred Helmholtz layer potential calculated from experimentalCEDL−VEDLdata and theoretical Hartree approximationCQ−VQ. The increase ofCHwith decreasing numbers of layers is evidence for correlations between electrode electrons and electrolyte ions that reduce the bias voltage necessary to drive charge transfer. Figure 4: EDL at the graphene/electrolyte interface. ( a ) Schematic illustration of the equivalent circuit and charge distribution near the graphene/electrolyte interface. ( b ) Quantum capacitance of graphene as a function of layer number and potential calculated in the standard self-consistent Hartree approximation which neglects correlations. Neglecting disorder, the carrier density in single-layer graphene is proportional to the square of the Fermi radius, and hence to square of the chemical potential. The capacitance is therefore linear in chemical potential. ( c ) Charge distribution induced at a potential of 0.1 V in graphene electrodes with different numbers of layers. Layer number 1 is exposed to the electrolyte. ( d ) Inferred Helmholtz capacitance plotted against inferred Helmholtz layer potential calculated from experimental C EDL − V EDL data and theoretical Hartree approximation C Q − V Q . The increase of C H with decreasing numbers of layers is evidence for correlations between electrode electrons and electrolyte ions that reduce the bias voltage necessary to drive charge transfer. Full size image Band theory calculation of graphene quantum capacitance Here we used a standard band theory calculation and note that, to the best of our knowledge, such a calculation for multilayer graphene is new. Figure 4b illustrates theoretical C Q values calculated as a function of the graphene potential V Q for graphene electrodes with different layer numbers. (Details of this model calculation are explained in Supplementary Note 4 and Supplementary Note 5 .) Note that C Q increases with layer number at all V Q even though charge is spread over more layers, and that it has a finite value of 2–4 μF cm −2 near V Q ~0 because of the finite temperature and disorder broadening effects [32] , [33] . The increase of C Q with layer number for a given V Q can be attributed to the increase of the DOS when more layers are added. However, this enhancement of the capacitance saturates quickly and the values of C Q for four- and five-layer graphene are almost identical. This is because the induced charge accumulates mainly on the outmost few layers (for example, n <5) that are close to the solid/liquid interface as a result of self-consistent electrostatic screening ( Fig. 4c ). However, the standard band theory calculation for an electrode without considering the electrolyte ( Fig. 4b ) cannot explain the anomalous capacitance decrease with the number of graphene layers ( Fig. 3 ) when our electrodes are charged. We attribute the enhanced capacitance we observe for single- and few-layer graphene electrodes to correlations between the π -band electron Fermi liquid and ions in the Helmholtz layer. These correlations can be discussed [34] , [35] in terms of attractive interactions between ions and image charges in the conducting graphene sheets that narrow the double layer, decrease the bias voltage necessary to drive charge separation and enhance the EDL capacitance. Our experiments suggest that correlations are more effective in enhancing capacitance when the number of graphene layers is reduced. The enhanced correlation can be captured in molecular dynamic (MD) simulations that account realistically for the response of graphene sheet electrons to ion locations. For bookkeeping purposes, we assign this contribution to the capacitance to C H . It is revealed most clearly when we use the theoretical quantum capacitances to extract C H −V H curves from experimental C EDL − V EDL data (details of the calculation are explained in Supplementary Fig. 8 and Supplementary Note 5 ). In Fig. 4d we see that C H increases substantially and becomes more dependent on V H with decreasing layer number. These effects are not ascribable to adsorption or faradic reaction of ions at the graphene surface as verified from the CV test ( Supplementary Fig. 5 ), and there is no sieving effect as in the case of nanopores, thus very likely, implying a stronger correlation between electrons in single-layer graphene and ions in electrolyte. A recent EDL capacitance study of a single-layer graphene in [BMIM][PF 6 ] ionic liquid interface [36] has shown that MD simulations can partly account for variations of Helmholtz capacitance C H not explained by commonly adopted assumptions. A complete understanding of the effects we observe will likely require the development of new calculation methods that account for the correlated response of carriers in the electrodes to ionic fluctuations. Our discovery of enhanced capacitance in extremely thin single-layer/multilayer graphene electrodes motivates further research on electrolyte–ions/electrode–electron correlations, and on ion packing on graphene and other 2D-material surfaces. From an experimental point of view, one approach is suggested by recent advances in the use of X-ray reflectivity to study spatial charge distributions in the liquid phase at the lipid/water interface [37] and at the charged/uncharged solid surface/ionic liquid interface [38] , [39] . These techniques could be used to probe the EDL at the interface between an ionic liquid and single-layer or multilayer graphene with spatial resolutions down to 0.3 nm. Other types of experiments which could be used to shed light on the EDL interface include electron energy loss spectroscopy in a scanning transmission electron microscope [40] and surface-enhanced Raman spectroscopy [41] . From the theoretical perspective, the substantial corrections to the capacitance values obtained from geometric considerations alone point to the importance of many-body effects influenced by electrode geometry and response properties for a complete understanding of energy storage at ionic liquid–electrode interfaces. Our findings pose an exciting theoretical challenge as they can only be accounted for using theories that go beyond conventional mean-field approximations and MD simulations which do not account for geometry-dependent electrode response properties. Further progress will require an interplay between theory and simulation, and experiments that provide detailed information on the spatial distribution of the electrolyte ions. Nevertheless, our calculation suggests that a low DOS of carbon electrodes at PZC suppresses capacitance, and the electrostatic correlation effects at higher carrier density enhance capacitance when the electrodes are charged. This speculation can be used, especially near the PZC, to conceptually interpret the non-rectangular shape of CV curves observed previously on some carbon electrodes consisting of single (or few)-layer graphene sheets, even when there is no pseudocapacitive contribution or ion-sieving effect in the systems [14] , [15] . Since single-layer graphene has no electrostatic screening effect that occurs in multilayer graphene, it has the strongest electrostatic correlation when the electrode is charged. Therefore, a single-layer graphene with improved DOS would be an excellent electrode candidate for EDL capacitors. Our experimental study on single-layer graphene electrodes with improved DOS achieved by nitrogen doping ( Supplementary Figs 9 , 10 and Supplementary Note 6 ) shows that the average capacitance over the total applied potential window of 0.4, 0.6 and 0.8 V, respectively, increases with the charge carrier density, n e . A maximum capacitance enhancement of 66% was reached by using nitrogen-doped single-layer graphene instead of pristine graphene (PG) ( Supplementary Fig. 10 and Supplementary Note 6 ), consistent with recently measured gravimetric capacitance improvements with nitrogen-doped carbon electrodes [21] . We have shown that the capacitances are anomalously enhanced for thicknesses below a few layers when the graphene sheets are charged, and ascribed it to a low DOS at the PZC which suppresses capacitance, and electrostatic correlation effects at higher carrier density which enhance capacitance. We anticipate that this result can trigger the development of new calculation methods in understanding the EDL at carbon/electrolyte interface. In addition, single-layer graphene has more prominent C EDL −V EDL response than multilayer graphene over the typical potential window for EDL capacitors with aqueous electrolytes. Since single-layer graphene has a SSA of 2630, m 2 g −1 , the area-normalized capacitance C EDL of 13.5 uF cm −2 (ref. 17 ) implies a gravimetric capacitance of 355 F g −1 . Assuming an optimized symmetric supercapacitor system in an organic electrolyte with a cell voltage of 4 V, we anticipate that the maximum limit of energy stored in a single-layer graphene-based supercapacitor could be as high as 59 Wh kg −1 . This energy density value is comparable to that of the lead-acid batteries in market, but with much higher power density and cycle stability because of the pure EDL energy storage mechanism. New classes of carbon, for example, ‘negative-curvature’ carbons [42] , which have higher theoretical SSA than normal porous carbons, with enhanced charge carrier density could take advantage of the mechanism discovered here. Synthesis and characterization of PG and NG PG and nitrogen-doped graphene (NG) were prepared on Cu by low-pressure chemical vapour deposition [26] , [43] , Typically, a 2 × 10 cm Cu stripe with thickness of 25 μm (99.8%, Alfa-Aesar, item No. 13382) was placed at the centre of a fused quartz tube with diameter of 2.5 cm that was heated in a split hot-wall furnace (TF55035A-1, Linderburg/Blue M). The tube was evacuated before ramping to 1,035 °C with 2 sccm hydrogen (99.999%, Airgas) flow at a pressure of 20 mtorr. The Cu foil was then annealed for 30 min under 2 sccm of hydrogen before introducing methane (99.999%, Airgas) and pyridine (>99.0%, Aldrich) mixture at different partial pressure ratios with total pressure of 70 mtorr at 1,035 °C for 7 min to make graphene with different nitrogen-doping levels. The partial pressure of hydrogen, methane and pyridine for PG and NG growth are summarized in Supplementary Table 1 . The numbers after ‘NG’ in Supplementary Table 1 stand for the fraction of the pyridine/methane partial pressure. The furnace was cooled down to room temperature at its natural cooling rate. The N dopant concentration was controlled by altering the ratio of partial pressures of methane and pyridine. Fabrication of graphene electrode The single-layer graphene on copper was transferred to a plastic substrate with partially dissolved copper as the electrical contact ( Fig. 1 ) for electrochemical measurements. First, one side of the graphene/copper was spin coated with PMMA (Aldrich), then, following route (1), scotch tape (3 M Corp.) with thickness of 85 μm was placed on the PMMA side. The single-layer graphene that was sandwiched between the scotch tape and copper was partially dipped in a 0.5 M ammonium persulphate (Aldrich) aqueous solution for dissolving the copper, which exposed the graphene to the solution and left the copper for electrical contact. The sample was rinsed with deionized water before electrochemical measurements in a 6 M KOH aqueous solution. Only pristine single-layer graphene was used for preparing multilayer graphene electrode, which was done by following route (2) after spin coating of PMMA. The copper was totally dissolved by ammonium persulphate aqueous solution then rinsed with deionized water before transferring the PMMA-coated graphene onto another piece of graphene-coated copper, which yielded two-layer graphene that was sandwiched between PMMA and copper. This process was repeated to obtain three, four and five layers of graphene, respectively. Then scotch tape was placed on the PMMA side before partially dissolving the copper for electrochemical measurements. Electrochemical measurements The EDL capacitance of graphene electrodes was measured in a 6 M KOH aqueous solution with a Pt plate (1.5 × 1.5 cm) as the counter electrode, a Ag/AgCl reference electrode (filled with 1 M KCl with potential of 0.236 V versus standard hydrogen electrode) and the graphene on tape as the working electrode. The copper did not touch the electrolyte during measurement to ensure that the electrochemical signal was generated at the graphene surface only. For each type of graphene electrodes that with different graphene layer numbers, we, respectively, measured 3–7 devices for statistical analysis. The electrochemical measurements were performed with an Eco Chemie Autolab PFSTAT100 potentiostat equipped with a FRA2 frequency response analyser module. CV at a scan rate of 20 mV s −1 was performed with each electrode to ensure only non-faradic activity occurs that there is no contamination existed at the graphene surface ( Supplementary Fig. 5 ). The capacitance was measured using electrode impedance spectroscopy. The electrode impedance spectroscopy was performed by using a sinusoidal signal with amplitude of 10 mV over a frequency range of 100 k−10 Hz and a scanning potential range of −0.7 to 0.5 V versus a Ag/AgCl reference electrode at a step size of 0.1 V. General characterization Scanning electron microscopy was carried out on FEI Quanta 600 (acceleration voltage of 30 kV for graphene on copper and of 2 kV for graphene electrodes). Micro-Raman was carried out on WITEC GmbH Alpha 300 (100 × 0.9 NA, objective lens and 488 nm laser excitation). X-ray photoemission spectroscopy was carried out on AXIS Ultra DLD system (equipped with a monochromatic Al Kα X-ray source (1486.6 eV)). How to cite this article: Ji, H. et al . Capacitance of carbon-based electrical double-layer capacitors. Nat. Commun. 5:3317 doi: 10.1038/ncomms4317 (2014).